The structure of the FANCM–MHF complex reveals physical features for functional assembly Fanconi anaemia is a rare genetic disease characterized by chromosomal instability and cancer susceptibility. The Fanconi anaemia complementation group protein M (FANCM) forms an evolutionarily conserved DNA-processing complex with MHF1/MHF2 (histone-fold-containing proteins), which is essential for DNA repair in response to genotoxic stress. Here we present the crystal structures of the MHF1–MHF2 complex alone and bound to a fragment of FANCM (FANCM 661−800 , designated FANCM-F). The structures show that MHF1 and MHF2 form a compact tetramer to which FANCM-F binds through a 'dual-V' shaped structure. FANCM-F and (MHF1–MHF2) 2 cooperate to constitute a new DNA-binding site that is coupled to the canonical L1L2 region. Perturbation of the MHF–FANCM-F structural plasticity changes the localization of FANCM in vivo . The MHF–FANCM interaction and its subcellular localization are altered by a disease-associated mutant of FANCM. These findings reveal the molecular basis of MHF–FANCM recognition and provide mechanistic insights into the pathway leading to Fanconi anaemia. The effective repair of DNA damage, caused by exogenous agents or arising during DNA replication, confers protection from malignant transformation. Several genetic disorders that perturb the repair of DNA damage result in an elevated predisposition to cancer. One such disorder is a rare, multigenic syndrome known as Fanconi anaemia (FA), which is characterized by developmental defects, bone marrow failure, and chromosomal instability [1] , [2] , [3] . Mutations in any of these 15 known FANC genes can result in dysfunctions in DNA damage repair, leading to FA [2] , [3] , [4] , [5] , [6] , [7] . FA cells are susceptible to agents that induce DNA interstrand crosslinks (ICLs), which block the progression of the replication fork. In response to DNA damage, FANCL in the FA core complex, composed of eight FA proteins (FANCA, -B, -C, -E, -F, -G, -L, and -M) [3] , monoubiquitinates the FANCD2–FANCI complex [8] , [9] . Once ubiquitinated, this complex recruits the downstream FA proteins, and the pathway for homologous recombination-dependent DNA repair is activated [10] . The recently identified FA-related protein, FAN1, may act as a direct effector, processing the ICL with its exonuclease activity on binding to ubiquitinated FANCD2–FANCI through its ubiquitin-binding zinc-finger domain [11] , [12] , [13] , [14] . As a component of the FA core complex, the Fanconi anaemia complementation group protein M (FANCM) contains an evolutionarily conserved helicase domain bearing ATP-dependent DNA translocase activity [15] , [16] , [17] . In addition to its interactions with other FA proteins [18] , FANCM possesses an activity for binding to branch-structured DNA [16] , which is required for efficient monoubiquitination of the FANCD2–FANCI heterodimer [19] . Recently, two histone-fold-containing proteins, MHF1 and MHF2, were identified as FANCM-associated factors [20] , [21] . The MHF1–MHF2 complex (abbreviated MHF) binds double-strand DNA (dsDNA) [20] , [21] , stimulates the DNA-binding activity of FANCM, and contributes to FANCM targeting to chromatin [21] . A stable association with FANCM and DNA-binding activity are required for MHF to function in activation of the FA pathway [20] , [21] . Moreover, like FANCM, MHF is conserved, from yeast to human [20] , [21] , suggesting the functional importance of the MHF–FANCM complex in eukaryotes. It is unclear, however, how FANCM physically interacts with MHF and whether the MHF–FANCM interaction is perturbed in the disease-associated mutant, FANCM S724X . In addition, MHF1 and MHF2 are constitutive, centromere-associated network proteins of CENP-S and CENP-X, which are implicated in assembly of the outer kinetochore [22] , [23] . However, it has remained to be determined whether CENP-S/X assembles into functional nucleosomes at the centromere and how those CENP-S/X-containing nucleosomes relate to the classical CENP-A-containing nucleosomes. Here we report the crystal structures of the MHF1–MHF2 complex alone and bound to FANCM 661−800 (FANCM-F). The structures show that MHF1 and MHF2 form a (MHF1–MHF2) 2 tetramer (MHF) and that FANCM-F binds to it through a 'dual-V' shaped structure. The (MHF1–MHF2) 2 tetramer cooperates with FANCM-F in DNA-binding through constructing an extra site on the complex. Perturbation of the MHF–FANCM-F interaction by FANCM S724X changes the FANCM localization in vivo , which suggests a potential mechanism underlying the pathogenesis of FA. Overall structure of MHF1–MHF2 complex To gain further insights into FA, we carried out structural studies on the MHF–FANCM complex. 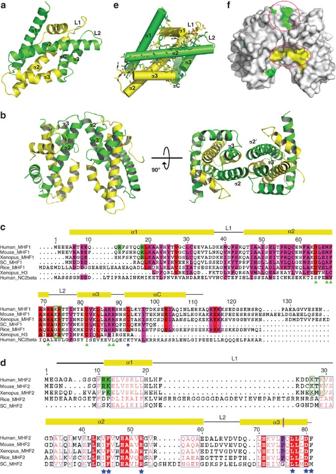Figure 1: Overall structure of the MHF complex. (a) Ribbon representation of the MHF1–MHF2 heterodimer. MHF1 and MHF2 are coloured in green and yellow, respectively, and the same colour style is used in the all subsequent figures, unless otherwise specified. Secondary structure element is termed based on that of Histones (see alsocandd). (b) Ribbon diagram of the (MHF1–MHF2)2tetramer. The right one is an orthogonal view from the top of the left one. (c) Sequence alignment of human MHF1 with mouse, Xenopus,Saccharomyces cerevisiae, and rice orthologues as well as H3 and NC2β. The identical and similar residues are depicted with red and magenta backgrounds, respectively. The residues, designated with a green triangle, are involved in the formation of (MHF1–MHF2)2tetramer. Residues labelled with a blue star reside in the MHF2 hydrophobic core. The residues in green backgrounds are located in the α1α1 site and those in green box are in the L1L2 site (see alsod). (d) Sequence alignment of human MHF2. The inserted Proline in the α3 is implicated with a green line. (e) MHF1–MHF2 dimer formation. Residues involved in the interactions are highlighted in green (MHF1) and yellow (MHF2) sticks. (f) Surface representation of (MHF1–MHF2)2tetramer coloured by sequence conservation. The mostly conserved residues in MHF1 are coloured in green and yellow for MHF2. Conserved residues form two clusters in three-dimensional space. Because full-length MHF1 in complex with MHF2 failed to yield crystals, truncated MHF1 with the carboxy-terminal 31 residues deleted was used for crystal growth and structure determination (Methods) ( Table 1 ). The structure shows that four MHF1–MHF2 heterodimers occupy the asymmetric unit ( Fig. 1a,b ), and they have an essentially identical structure, as revealed by structural superposition (0.69 Å RMSD). In addition to the three central α helices for MHF1 and MHF2, an extra C-terminal αC helix is included in MHF1 ( Fig. 1a–d ). The MHF1–MHF2 heterodimer is mediated by the histone-fold in a head-to-tail fashion, commonly found in histone-like proteins [24] , [25] , [26] . Numerous hydrophobic and polar contacts occur at the dimer interface and result in a buried surface area of about 2,245 Å 2 ( Fig. 1e ), which is consistent with their stable association during the purification process. MHF1 uses its C-terminal parts of α2 and α3 to assemble into a (MHF1–MHF2) 2 tetramer, constructing a four-helix bundle with a pseudodyad passing across the interface ( Fig. 1b ; Supplementary Fig. S1 ), as occurs for (H3–H4) 2 and (CENP-A-H4) 2 (refs 27 , 28 ). Table 1 Data collection and refinement statistics. Full size table Figure 1: Overall structure of the MHF complex. ( a ) Ribbon representation of the MHF1–MHF2 heterodimer. MHF1 and MHF2 are coloured in green and yellow, respectively, and the same colour style is used in the all subsequent figures, unless otherwise specified. Secondary structure element is termed based on that of Histones (see also c and d ). ( b ) Ribbon diagram of the (MHF1–MHF2) 2 tetramer. The right one is an orthogonal view from the top of the left one. ( c ) Sequence alignment of human MHF1 with mouse, Xenopus, Saccharomyces cerevisiae , and rice orthologues as well as H3 and NC2β. The identical and similar residues are depicted with red and magenta backgrounds, respectively. The residues, designated with a green triangle, are involved in the formation of (MHF1–MHF2) 2 tetramer. Residues labelled with a blue star reside in the MHF2 hydrophobic core. The residues in green backgrounds are located in the α1α1 site and those in green box are in the L1L2 site (see also d ). ( d ) Sequence alignment of human MHF2. The inserted Proline in the α3 is implicated with a green line. ( e ) MHF1–MHF2 dimer formation. Residues involved in the interactions are highlighted in green (MHF1) and yellow (MHF2) sticks. ( f ) Surface representation of (MHF1–MHF2) 2 tetramer coloured by sequence conservation. The mostly conserved residues in MHF1 are coloured in green and yellow for MHF2. Conserved residues form two clusters in three-dimensional space. Full size image Structural features of MHF1–MHF2 complex Although MHF1/MHF2 belongs to H2A/H2B family owing to the existence of MHF1 αC helix, MHF1 preserves the partial feature of H3/H4, evident by the presence of an intra-chain arginine-aspartate bidentate pair observed in H3/H4 and NC-Y [24] , [27] . MHF1 residues, Arg73 and Asp81, conserved across species ( Fig. 1c ), interact electrostatically with each other, whereas MHF2 Arg64 is positioned too close to Asp66 to form that kind of bidentate ( Fig. 2a–c ). MHF1–MHF2 and H2A–H2B heterodimers superimpose with a 2.46-Å RMSD over Cα atoms, located in histone-fold regions. A corresponding MHF1–MHF2 and H3–H4 superposition has a 1.88-Å RMSD. Significant structural differences between MHF1/MHF2 and H2A/H2B reside in the amino terminus of MHF1 and C terminus of MHF2. MHF1 lacks the N-terminal extension as that of H2B, but processes a longer α1 helix ( Fig. 2d ); MHF2 does not contain extra C-terminal helix and tail ( Fig. 2a ). Further, the MHF2 α3 helix adopts a different conformation and it is more bent towards α2 ( Fig. 2e ). There are two reasons for the helix kink. First, the insertion of Pro75 into the primary sequence destroys the continuation of the α3 helix ( Fig. 2e ). Second, the hydrophobic core, comprised of MHF1 Leu92, MHF2 Val44, Phe45, Leu77, Phe81, as well as intra-chain electrostatic contacts between MHF2 Arg52 and Asp80, restrains the local conformation ( Fig. 2e ). Notably, the residues participating in above interactions are highly conserved across species ( Fig. 1c–f ). 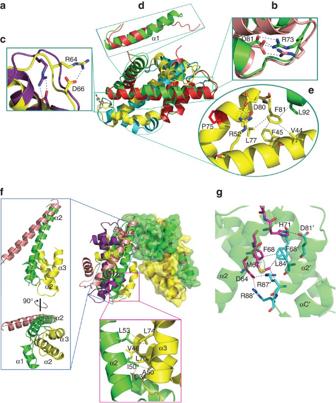Figure 2: Structural comparisons of MHF with histone-fold proteins. (a) Comparisons of MHF with histones from nucleosome (PDB ID: 1AOI). H2A was in cyan, H2B in red, H3 in salmon and H4 in violet purple. The (b) close-up view highlights the Arg–Asp bidentate pair of MHF1. The (c) clos-eup view shows that MHF2 does not contain the bidentate pair. The (d) close-up view illustrates the difference of α1 helix in MHF1 and H2B. The (e) close-up view reveals the local environment causing the α3 kink of MHF2. (f) Overlay of (MHF1–MHF2)2with (H3–H4)2. The dimer used for alignment is shown in a surface representation. The left close-up view highlights the α2 helix conformation and the bottom close-up view reveals the hydrophobic interactions. The trajectory of α2 helix was modelled with black dashes. (g) The specific interface of (MHF1–MHF2)2tetramer. Residues participating in the interactions are shown in magenta sticks for one MHF1 molecule and cyan sticks for the pseudo-symmetry-related MHF1′. Figure 2: Structural comparisons of MHF with histone-fold proteins. ( a ) Comparisons of MHF with histones from nucleosome (PDB ID: 1AOI). H2A was in cyan, H2B in red, H3 in salmon and H4 in violet purple. The ( b ) close-up view highlights the Arg–Asp bidentate pair of MHF1. The ( c ) clos-eup view shows that MHF2 does not contain the bidentate pair. The ( d ) close-up view illustrates the difference of α1 helix in MHF1 and H2B. The ( e ) close-up view reveals the local environment causing the α3 kink of MHF2. ( f ) Overlay of (MHF1–MHF2) 2 with (H3–H4) 2 . The dimer used for alignment is shown in a surface representation. The left close-up view highlights the α2 helix conformation and the bottom close-up view reveals the hydrophobic interactions. The trajectory of α2 helix was modelled with black dashes. ( g ) The specific interface of (MHF1–MHF2) 2 tetramer. Residues participating in the interactions are shown in magenta sticks for one MHF1 molecule and cyan sticks for the pseudo-symmetry-related MHF1′. Full size image Structural superimposition of one MHF1–MHF2 heterodimer to that of (H3–H4) 2 reveals that the (MHF1–MHF2) 2 tetramer adopts a highly compact structure ( Fig. 2f ). First, the bent of MHF1 α2 helix towards MHF2 induced by the hydrophobic interactions positioned in the N-terminal part of the MHF1 α2 helix gives a close proximity ( Fig. 2f ). Second, the rotation between the dimer pairs of (MHF1–MHF2) 2 relative to that of (H3–H4) 2 further tightens the tetramer ( Fig. 2f ). A series of hydrophobic and polar contacts within the four-helix bundle interface maintains the rotation divergence. In addition to the hydrogen bonds between His71 and Asp81′, which is conserved in (H3–H4) 2 , the hydrophobic interaction, mediated by the aliphatic side of Met67, and aromatic ring of Phe68 stabilizes the tetramer ( Figs 1c and 2g ). Notably, Arg87′ not only participates in the hydrophobic interaction, through aliphatic portion of side chain, but, together with Arg88′, also forms ion pairs with Asp64 ( Fig. 2g ). These ion pairs, positioned further away from the top interactions, thus contribute to a specialized α2–α2′ conformation. In sum, our structural observations reveal that MHF1 and MHF2 form a compact tetramer. FANCM binds to the (MHF1–MHF2) 2 tetramer FANCM was previously found to associate with MHF1–MHF2 through the region consisting of residues 661–800 (ref. 21 ). We co-crystallized the FANCM fragment (FANCM 661–800 , designated FANCM-F) with MHF1–MHF2 and determined the structure of the complex ( Table 1 ). The structure shows that one FANCM-F molecule binds to a (MHF1–MHF2) 2 tetramer and that FANCM-F exhibits an extended conformation ( Fig. 3a,b ). The binding of FANCM-F to a pseudodyad-related (MHF1–MHF2) 2 tetramer results in a pseudo-two-fold symmetric shape of FANCM-F, like two 'V's connected by a linker coil passing through the interspace formed by the two α3 helices of MHF2/MHF2′. Without association with MHF, FANCM-F seems to be disordered in solution, as the residues that do not participate in the interaction with MHF, including the N- and C-terminal FANCM-F and residues 730–50, either have no electron density or are highly flexible ( Fig. 3c,d ). The ordered portion of FANCM-F, folding into three α helices and irregular coil with elements of two small β-strands and two 3 10 helices, remains in almost continuous contact with (MHF1–MHF2) 2 through wrapping around the MHF1 α1, α2 and MHF2 α2, α3 helices ( Fig. 3a,b ). 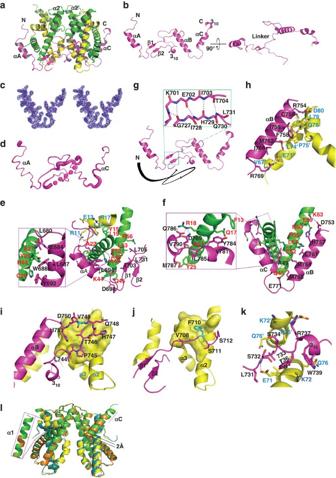Figure 3: FANCM-F binds to (MHF1–MHF2)2tetramer. (a) Ribbon representation of the overall structure of MHF–FANCM-F complex, with FANCM-F in magenta. The dimer associating with the N-terminal part of FANCM-F is labelled as MHF and the other one, interacting with the FANCM-F C terminus, is labelled as MHF′. (b) The extended structure of FANCM-F. (c) Representative experimental electron density map. Electron density map at 2.64 Å resolution contoured at 1.0 σ. The portion of FANCM-F residues 753–86 is shown. (d) The B-factor distribution of FANCM-M. The wider the tubing is, the higher the B-factor. The missing residues 730–50 are modelled in magenta circles. (e) The N-terminal 'V' segment wraps around the MHF1 α1 and α2 helices. Close-up view indicates the complementary hydrophobic interface between FANCM-F αA and MHF1 α1 helix. The involved residues are labelled in black, red and blue letters for FANCM-F, MHF1 and MHF2, respectively. (f) The C-terminal 'V' segment surrounds the same region of MHF1′ as ine. (g) The β2 strand forms five hydrogen bonds with β1. The black arcuate line indicates the trajectory of FANCM-F. (h) FANCM-F αB helix packs against α3/α3′ of MHF2/MHF2′. (i) The coil covers the surface area of partial α2′ and α3′ of MHF2′. Residues shown in sticks all make contacts with MHF2. Val749 highlighted in cyan stick inserts its side chain into the MHF2 hydrophobic core. (j) The coil following α1 extends to Gln714. FANCM-F Phe710 interacts with the MHF2 hydrophobic core with the aromatic ring. (k) The linker coil interacts with the bottom parts of MHF2 α3, viewed from the bottom in (i). (l) Structure comparison of the two (MHF1–MHF2)2tetramers. MHF1 and MHF2 from the MHF complex are shown in orange and deep teal, respectively; those from the FANCM-F bound are shown green (MHF1) and yellow (MHF2), respectively. The line and the boxes indicate the region where difference occurs. Figure 3: FANCM-F binds to (MHF1–MHF2) 2 tetramer. ( a ) Ribbon representation of the overall structure of MHF–FANCM-F complex, with FANCM-F in magenta. The dimer associating with the N-terminal part of FANCM-F is labelled as MHF and the other one, interacting with the FANCM-F C terminus, is labelled as MHF′. ( b ) The extended structure of FANCM-F. ( c ) Representative experimental electron density map. Electron density map at 2.64 Å resolution contoured at 1.0 σ. The portion of FANCM-F residues 753–86 is shown. ( d ) The B-factor distribution of FANCM-M. The wider the tubing is, the higher the B-factor. The missing residues 730–50 are modelled in magenta circles. ( e ) The N-terminal 'V' segment wraps around the MHF1 α1 and α2 helices. Close-up view indicates the complementary hydrophobic interface between FANCM-F αA and MHF1 α1 helix. The involved residues are labelled in black, red and blue letters for FANCM-F, MHF1 and MHF2, respectively. ( f ) The C-terminal 'V' segment surrounds the same region of MHF1′ as in e . ( g ) The β2 strand forms five hydrogen bonds with β1. The black arcuate line indicates the trajectory of FANCM-F. ( h ) FANCM-F αB helix packs against α3/α3′ of MHF2/MHF2′. ( i ) The coil covers the surface area of partial α2′ and α3′ of MHF2′. Residues shown in sticks all make contacts with MHF2. Val749 highlighted in cyan stick inserts its side chain into the MHF2 hydrophobic core. ( j ) The coil following α1 extends to Gln714. FANCM-F Phe710 interacts with the MHF2 hydrophobic core with the aromatic ring. ( k ) The linker coil interacts with the bottom parts of MHF2 α3, viewed from the bottom in ( i ). ( l ) Structure comparison of the two (MHF1–MHF2) 2 tetramers. MHF1 and MHF2 from the MHF complex are shown in orange and deep teal, respectively; those from the FANCM-F bound are shown green (MHF1) and yellow (MHF2), respectively. The line and the boxes indicate the region where difference occurs. Full size image The MHF1–FANCM-F interaction is characterized by the pseudo-symmetry with each 'V' segment and the associated MHF1–MHF2 dimer as a subregion. FANCM-F αA helix spans MHF1 α1 and makes interactions by forming a complementary hydrophobic interface consisting of FANCM-F residues Leu680, Glu684, Leu687, Trp688 and Tyr692, and MHF1 residues Ala21, Ala22, His24, Tyr25 and Cys29 ( Fig. 3e ). Accordingly, FANCM-F αC, together with the following 3 10 helix and 3-residue linker, surrounds the same region of MHF1′ on the other side, which involves FANCM-F residues Val781, Tyr784, Leu785, Met787 and Val790 ( Fig. 3f ). MHF1′ residue Arg18′ forms 3 hydrogen bonds with Gln786 and Asp789 of FANCM-F through side chain ( Fig. 3f ). Following αA, β1 is kept in position through hydrophobic interactions between FANCM-F residues Leu694, Ile703, Leu705 and Leu731, and MHF1 residues Gln45, Ala48, Ala49, Glu52, Leu53 and Arg56, located within the N terminus of α2 ( Fig. 3e ). Notably, the FANCM-F residues 727-30, making five pairs of hydrogen bonds with β1, fold into the β2 strand, which is used to rotate the polypeptide for the arrival at the other side of the tetramer ( Fig. 3g ). The FANCM-F αB helix, equivalent to the β1 strand, packs against the MHF1′ α2′ helix in an anti-parallel manner, with its hydrophobic side facing α2′ ( Fig. 3f ). FANCM-F αB helix and the linker coil are the main elements constructing the MHF2–FANCM-F interface, which buries a total surface area of about 2,161 Å 2 . Besides the contacts with MHF1, FANCM-F αB also packs against the two α3 helices of MHF2/MHF2′, generating hydrophobic interactions as well as 3 hydrogen bonds together with the flanking Arg769 ( Fig. 3h ). The coil immediately N-terminal to the FANCM-F αB, sticks to the surface created by MHF2 α2′ and α3′, thus preventing the MHF2 hydrophobic coil from solvent access ( Fig. 3i ). The N-terminal counterpart coil lacks the broad interface, but an aromatic residue Phe710, instead of the equivalent Val749, is used to interact with the MHF2 hydrophobic core ( Fig. 3i,j ). The loop and following 3 10 helix passing across the interspace of the two α3 helices of MHF2/MHF2′ further occlude the MHF2 hydrophobic core at the bottom through a series of interactions, among which FANCM-F Trp736 and Trp739 embedding the aliphatic portion of MHF2 Lys72 side chain stands out ( Fig. 3k ). The extensive buried surface area of about 4,328 Å 2 between MHF and FANCM-F explains their stable association in vivo [20] , [21] . The (MHF1–MHF2) 2 tetramer from the MHF–FANCM-F bears a similar structure as that of MHF complex alone (0.87 Å RMSD). The main differences between the two structures reside in the N and C termini of MHF1/MHF1′. For MHF1 in MHF–FANCM-F, αC not only becomes longer, but also moves about 2 Å towards FANCM-F ( Fig. 3l ). For MHF1′, α1′ becomes two turns longer with the extra traced residues ( Fig. 3l ). Both the C-terminal parts of α2 and α2′ in MHF2/MHF2′ are slightly bent away from the position in the MHF complex alone ( Fig. 3l ). In summary, (MHF1–MHF2) 2 tetramer retains the rigid structure and interface on binding with FANCM-F. Centromere localization of the (MHF1–MHF2) 2 tetramer As observed above, the finding of compact (MHF1–MHF2) 2 tetramer being retained in MHF–FANCM-F complex prompted us to speculate that the structural rigidity of (MHF1–MHF2) 2 is required for its in vivo function. To test the hypothesis, we generated two MHF1 mutants that were designed to disrupt the four-helix bundle: MHF1 D64A/F68A and MHF1 H71A/D81A ( Supplementary Fig. S1 ). Consistent with the structural observation, immunoprecipitation results showed that both Flag-tagged MHF1 mutants were incapable of associating with GFP-tagged MHF1 ( Fig. 4a ). Although wild-type MHF1 localized to the centromere marked by ACA (anti-centromere antibody, Fig. 4b ), the MHF1 H71A/D81A mutant failed to localize properly, suggesting that functional assembly of MHF1 dimer is essential for proper targeting and/or stable localization ( Fig. 4b ). In fact, the previous study has shown that MHF1 R87A/R88A , where mutations again are involved in the four-helix bundle interface, exhibits functional defects in activation of the FA pathway [21] . To destabilize the fold of the tetramer, we destroyed the MHF2 hydrophobic core by mutating the last two residues (Asp80/Phe81) of MHF2 into alanines (MHF2 D80A/F81A ) ( Supplementary Fig. S1 ). As anticipated, the mutant failed to localize to the centromere ( Fig. 4c ). Although MHF2 residues Asp80 and Phe81 do not participate in the direct physical contact with MHF1, the association between MHF1 and MHF2 was perturbed by their mutations ( Fig. 4d ). Moreover, MHF1 residues, Asp64, Phe68, His71, Asp81, Arg87 and Arg88, that are not in direct contact with MHF2 are important for MHF2 binding as well as for FANCM association in vivo [21] . These data suggest that assembly of the functional MHF–FANCM complex depends on the structural integrity of each unit and that the integrity of (MHF1–MHF2) 2 is essential for its distribution and function in cell culture. 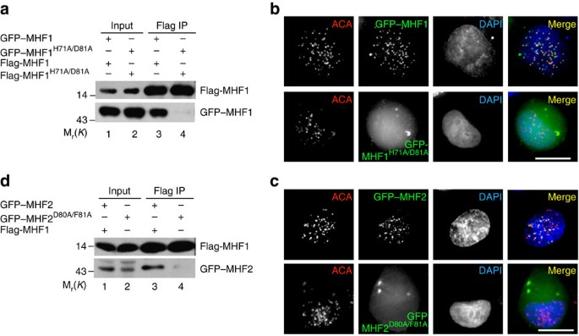Figure 4: Formation of the (MHF1–MHF2)2tetramer is essential for MHF functionin vivo. (a) Dimeric complex of MHF1 is disrupted by His71A and Asp81A mutations. Immunoprecipitation results show that wild-type Flag-MHF1 pulls down GFP–MHF1 (lane 3) but not MHF1H71A/D81Amutant (lane 4). (b) (MHF1–MHF2)2tetramer is essential for a stable localization to centromere. GFP–MHF1 is readily apparent as it co-localizes with centromere mark ACA (anti-centromere autoantibody; upper panel merge). GFP–MHF1H71A/D81Afailed to localize to the centromere as the GFP signal was not concentrated to the centromere (lower panel). (c) Integral (MHF1–MHF2)2is essential for a stable localization to centromere. GFP–MHF2 is readily apparent as it colocalizes with centromere mark ACA (upper panel merge). GFP–MHF2D80A/F81Afailed to localize to the centromere as the GFP signal was not concentrated to the centromere (lower panel). (d) MHF1–MHF2 heterodimer is perturbed by mutation of MHF2D80A/F81A. Western blot analysis results show that MHF1 pulls down GFP–MHF2 (lane 3) but not MHF2D80A/F81Amutant (lane 4). Figure 4: Formation of the (MHF1–MHF2) 2 tetramer is essential for MHF function in vivo . ( a ) Dimeric complex of MHF1 is disrupted by His71A and Asp81A mutations. Immunoprecipitation results show that wild-type Flag-MHF1 pulls down GFP–MHF1 (lane 3) but not MHF1 H71A/D81A mutant (lane 4). ( b ) (MHF1–MHF2) 2 tetramer is essential for a stable localization to centromere. GFP–MHF1 is readily apparent as it co-localizes with centromere mark ACA (anti-centromere autoantibody; upper panel merge). GFP–MHF1 H71A/D81A failed to localize to the centromere as the GFP signal was not concentrated to the centromere (lower panel). ( c ) Integral (MHF1–MHF2) 2 is essential for a stable localization to centromere. GFP–MHF2 is readily apparent as it colocalizes with centromere mark ACA (upper panel merge). GFP–MHF2 D80A/F81A failed to localize to the centromere as the GFP signal was not concentrated to the centromere (lower panel). ( d ) MHF1–MHF2 heterodimer is perturbed by mutation of MHF2 D80A/F81A . Western blot analysis results show that MHF1 pulls down GFP–MHF2 (lane 3) but not MHF2 D80A/F81A mutant (lane 4). Full size image L1L2 and the C-terminal MHF1 is necessary for MHF DNA-binding The DNA-binding activity of the MHF complex is necessary for its functions in cell culture, including FANCD2 monoubiquitination and suppression of sister-chromatid exchanges [20] , [21] . As occurs for (H3–H4) 2 , the calculated electrostatic surface potential of (MHF1–MHF2) 2 tetramer shows a positive charge on the convex side ( Fig. 5a,b ), which is probably involved in DNA-binding. By superimposing the MHF1–MHF2 dimer onto H2A–H2B from nucleosomes or NC2α–NC2β [25] , [26] , we concluded that the bound DNA fragment on the (MHF1–MHF2) 2 tetramer would follow a similar trajectory as that complexed with H2A–H2B or NC2α–NC2β ( Fig. 3c,d ), and L1L2 (the region composed by MHF1 L2 loop and MHF2 L1 loop; Fig. 1 ) is the DNA-binding site of (MHF1–MHF2) 2 , which is consistent with the amino-acid conservation in L1L2 ( Fig. 1c,d ). 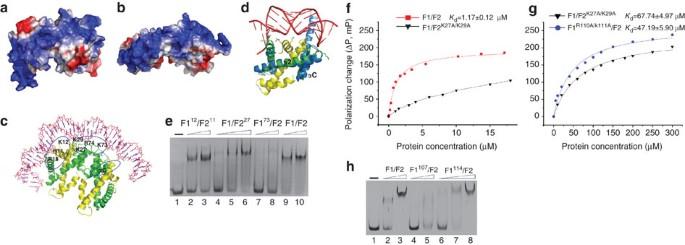Figure 5: The MHF complex has DNA-binding activity. Calculated electrostatic on the surface of (MHF1–MHF2)2tetramer (a) and (H3–H4)2from nucleosome (PDB ID: 1AOI) (b). Red and blue surfaces represent negative and positive electrostatic potentials (−3.5 kBT, +3.5 kBT), respectively. The electrostatic potentials were calculated using the Adaptive Poisson-Boltzmann Solver (APBS) with PyMol APBS tools. (c) Model of (MHF1–MHF2)2bound to DNA. Nucleosomal DNA was docked onto (MHF1–MHF2)2tetramer through alignment of MHF1–MHF2 dimer with H2A–H2B (PDB ID: 1AOI). The left blue circle indicates the α1α1 site, the middle one for L1L2 site and the right one for MHF1 C terminus. (d) L1L2 site and αC helix would face the bound DNA modelled by alignment of MHF1 with NC2α (blue). (e) EMSA results of MHF1–MHF2 complex and the mutants. 0.6 μM DNA substrate (59 bp, Methods); proteins at lanes 1–3 (MHF1R12A/R18A/MHF2R11A/K12A): 0, 5, 10 μM, respectively; lanes 4–6 (MHF1/MHF2K27A/K29A): 5, 10, 20 μM, respectively; lanes 7–8 (MHF1K73A/R74A/MHF2): 10, 20 μM, respectively; lanes 9–10 (MHF1/MHF2): 5, 10 μM, respectively. (f) FPAs of MHF1/MHF2 and MHF1/MHF2K27A/K29A. The data of wild-type MHF was fitted according to equation (2) (Methods). (g) FPAs of mutant MHF complexes, MHF1/MHF2K27A/K29Aand MHF1R110A/K111A/MHF2. (h) The DNA-binding effect of C terminus deletion on MHF1. 0.6 μM DNA substrate; proteins at lanes (MHF1/MHF2) 1–3: 0, 5, 10 μM; lanes 4–5 (MHF11−107/MHF2): 20 μM, 50 μM; lanes 6–8 (MHF11−114/MHF2): 5, 20, 50 μM, respectively. Figure 5: The MHF complex has DNA-binding activity. Calculated electrostatic on the surface of (MHF1–MHF2) 2 tetramer ( a ) and (H3–H4) 2 from nucleosome (PDB ID: 1AOI) ( b ). Red and blue surfaces represent negative and positive electrostatic potentials (−3.5 k B T, +3.5 k B T), respectively. The electrostatic potentials were calculated using the Adaptive Poisson-Boltzmann Solver (APBS) with PyMol APBS tools. ( c ) Model of (MHF1–MHF2) 2 bound to DNA. Nucleosomal DNA was docked onto (MHF1–MHF2) 2 tetramer through alignment of MHF1–MHF2 dimer with H2A–H2B (PDB ID: 1AOI). The left blue circle indicates the α1α1 site, the middle one for L1L2 site and the right one for MHF1 C terminus. ( d ) L1L2 site and αC helix would face the bound DNA modelled by alignment of MHF1 with NC2α (blue). ( e ) EMSA results of MHF1–MHF2 complex and the mutants. 0.6 μM DNA substrate (59 bp, Methods); proteins at lanes 1–3 (MHF1 R12A/R18A /MHF2 R11A/K12A ): 0, 5, 10 μM, respectively; lanes 4–6 (MHF1/MHF2 K27A/K29A ): 5, 10, 20 μM, respectively; lanes 7–8 (MHF1 K73A/R74A /MHF2): 10, 20 μM, respectively; lanes 9–10 (MHF1/MHF2): 5, 10 μM, respectively. ( f ) FPAs of MHF1/MHF2 and MHF1/MHF2 K27A/K29A . The data of wild-type MHF was fitted according to equation (2) (Methods). ( g ) FPAs of mutant MHF complexes, MHF1/MHF2 K27A/K29A and MHF1 R110A/K111A /MHF2. ( h ) The DNA-binding effect of C terminus deletion on MHF1. 0.6 μM DNA substrate; proteins at lanes (MHF1/MHF2) 1–3: 0, 5, 10 μM; lanes 4–5 (MHF1 1−107 /MHF2): 20 μM, 50 μM; lanes 6–8 (MHF1 1−114 /MHF2): 5, 20, 50 μM, respectively. Full size image Consistent with the structural analyses, MHF1 K73A/R74A exhibits diminished DNA-binding activity [21] ( Fig. 5e ). Similarly, as shown in Fig. 5e–g , MHF2 K27A/K29A exhibits a reduced binding affinity to dsDNA, judged by a significant increase in the dissociation constant ( K d ). Several residues in α1α1 of H2A–H2B from nucleosome or NC2α–NC2β are in direct contact with DNA [26] , [27] , thus contributing to the stability of the DNA-protein complex. However, the basic amino acids in the α1α1 of MHF seem to be dispensable in DNA-binding, as the combination mutant of MHF1 R12A/R18A and MHF2 R11A/K12A exhibits a slightly reduced DNA-binding affinity relative to the wild-type protein ( Fig. 5e ). Although the double-mutant associates with dsDNA, we could not rule out the possibility that the MHF basic residues in α1α1 make contacts with DNA, when the substrate is bound on the MHF. The likely reason that MHF1 R12A/R18A and MHF2 R11A/K12A mutations have little influence on the DNA-binding activity is that the L1L2 site alone is strong enough to support DNA-binding. The C terminus of MHF1 is indispensable for the DNA-binding activity of the MHF complex [20] . We confirmed the result by using the truncated complex for structure determination ( Fig. 3h ). Consistent with the previous observation, a 7-residue extension at the C terminus of the above truncation restored the DNA-binding activity, although with slightly lower affinity compared with the wild-type complex ( Fig. 3h ). MHF1 R110A/K111A in complex with MHF2 also exhibited a decreased DNA-binding affinity ( Fig. 3g ). Although the C terminus of MHF1 is predicted to be flexible and is not included in our structure, it may become ordered when associating with DNA substrate, as speculated from alignment of MHF1–MHF2 with NC2α–NC2β ( Fig. 3d ). We conclude that both the L1L2 site and C-terminal MHF1 are the molecular determinants for MHF1–MHF2 complex binding to DNA. MHF cooperates with FANCM-F in promoting DNA-binding Previous studies have revealed that FANCM stimulates the DNA-binding activity of MHF and vice versa [21] . As mentioned above, no structural allosterism is observed for the (MHF1–MHF2) 2 tetramer on FANCM-F binding; however, its electrostatic surface potential is changed. As shown in Fig. 6a,b , the α1α1 area of MHF–FANCM-F becomes more electropositive and broader than that of MHF alone because of the addition of FANCM-F N-terminal residues Lys675, Lys676, Lys686, Arg690 and Arg693, while the positive charge of the α1′α1′ site is neutralized by the Glu and Asp residues present at the C terminus of FANCM-F. When we analysed the DNA-binding profile of MHF–FANCM-F by fluorescence polarization assay (FPA), the two-site-binding mode was needed to fit the experimental data, which is different from the one-site-binding mode of MHF complex alone ( Figs 5f and 6c ). Surprisingly, the calculated K d 1 for MHF–FANCM-F is about tenfold lower than that of MHF ( Figs 5f and 6c ). This is reminiscent of the DNA-binding synergy between MHF and FANCM. Thus, we reasoned that MHF α1α1 and FANCM-F N terminus cooperate to create a new DNA-binding site (designated as the α1α1 site) on formation of a MHF–FANCM-F complex, in addition to the canonical L1L2 site. If this were the case, MHF–FANCM-F complex would still possess a DNA-binding property, even if MHF were in mutant form: MHF1 K73A/R74A /MHF2 or MHF1/MHF2 K27A/K29A . Indeed, our electrophoretic mobility shift assay (EMSA) results showed that MHF1 K73A/R74A /MHF2/FANCM-F interacts with DNA and that MHF1/MHF2 K27A/K29A /FANCM-F acts in a similar manner ( Fig. 6d ). We then determined whether mutations in the N terminus of FANCM-F would disrupt the α1α1 site by constructing two FANCM-F mutants: FANCM-F K675A/K676A and FANCM-F K686A/R690A/R693A . MHF1 K73A/R74A /MHF2/FANCM-F K675A/K676A lost the DNA-binding activity, and MHF1 K73A/R74A /MHF2/FANCM-F K686A/R690A/R693A showed defects in DNA-binding ( Fig. 6e ). Moreover, when FANCM-F K686A/R690A/R693A was complexed with MHF bearing MHF1 R12A/R18A/K73A/R74A mutations, it completely lost DNA-binding activity ( Fig. 6e ). Similarly, when FANCM-F K675A/K676A was complexed with MHF1 K73A/R74A and MHF2 R11A/K12A , any unspecific background was eliminated ( Fig. 6e ). 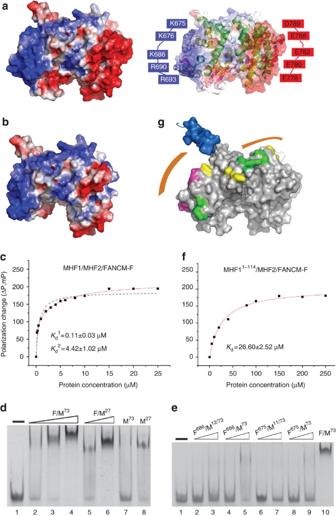Figure 6: MHF–FANCM-F complex possesses two DNA-binding sites. (a) Calculated electrostatic on the surface of (MHF1–MHF2)2bound to FANCM-F. Although some of the labelled residues shown in spheres (right one) having missing atoms in the final model, intact residues rebuilt in COOT were used for surface potential calculation. As a control, the surface potential of (MHF1–MHF2)2alone are shown in (b). Red and blue surfaces represent negative and positive electrostatic potentials (−3.5 kBT, +3.5 kBT). (c) FPA of MHF1/MHF2/FANCM-F. The data was fitted according to equation (3) (Methods). Blue dashes represent the results of data fitting according to equation (2) . Clearly, it is largely divergent from the experimental data. (d) EMSA results of the FANCM-F in complex with MHF mutants. 0.6 μM DNA substrate; proteins at lanes 1–4 (MHF1K73A/R74A/MHF2/FANCM-F): 0, 5, 10, 20 μM, respectively; lanes 5–6 (MHF1/MHF2K27A/K29A/FANCM-F): 5, 20 μM, respectively; lane 7 (MHF1K73A/R74A/MHF2): 20 μM; lane 8 (MHF1/MHF2K27A/K29A): 20 μM. (e) EMSA results of the FANCM-F mutants in complex with MHF mutants. 0.6 μM DNA substrate; proteins at lanes 1–3 (MHF1R12A/R18A/K73A/R74A/MHF2/FANCM-FK686A/R690A/R693A): 0, 5, 20 μM, respectively; lanes 4–5 (MHF1K73A/R74A/MHF2/FANCM-FK686A/R690A/R693A): 5, 20 μM, respectively; lane 6-7 (MHF1K73A/R74A/MHF2R11A/K12A/FANCM-FK675A/K676A), 5, 20 μM; lane 8-9 (MHF1K73A/R74A/MHF2/FANCM-FK675A/K676A): 5, 20 μM, respectively; lane 10 (MHF1K73A/R74A/MHF2/FANCM-F): 20 μM. (f) MHF11−114/MHF2/FANCM-F still binds to DNA. But the data could only be fitted in one-site-binding mode. (g) The DNA-binding trajectory in the MHF–FANCM-F complex. MHF1 C terminus locates in the junction of the two DNA-binding paths shown in orange strip, and the MHF1 C-terminal residues may follow a trajectory similar to that of α4 helix of NC2α shown in blue. Figure 6: MHF–FANCM-F complex possesses two DNA-binding sites. ( a ) Calculated electrostatic on the surface of (MHF1–MHF2) 2 bound to FANCM-F. Although some of the labelled residues shown in spheres (right one) having missing atoms in the final model, intact residues rebuilt in COOT were used for surface potential calculation. As a control, the surface potential of (MHF1–MHF2) 2 alone are shown in ( b ). Red and blue surfaces represent negative and positive electrostatic potentials (−3.5 k B T, +3.5 k B T). ( c ) FPA of MHF1/MHF2/FANCM-F. The data was fitted according to equation (3) (Methods). Blue dashes represent the results of data fitting according to equation (2) . Clearly, it is largely divergent from the experimental data. ( d ) EMSA results of the FANCM-F in complex with MHF mutants. 0.6 μM DNA substrate; proteins at lanes 1–4 (MHF1 K73A/R74A /MHF2/FANCM-F): 0, 5, 10, 20 μM, respectively; lanes 5–6 (MHF1/MHF2 K27A/K29A /FANCM-F): 5, 20 μM, respectively; lane 7 (MHF1 K73A/R74A /MHF2): 20 μM; lane 8 (MHF1/MHF2 K27A/K29A ): 20 μM. ( e ) EMSA results of the FANCM-F mutants in complex with MHF mutants. 0.6 μM DNA substrate; proteins at lanes 1–3 (MHF1 R12A/R18A/K73A/R74A /MHF2/FANCM-F K686A/R690A/R693A ): 0, 5, 20 μM, respectively; lanes 4–5 (MHF1 K73A/R74A /MHF2/FANCM-F K686A/R690A/R693A ): 5, 20 μM, respectively; lane 6-7 (MHF1 K73A/R74A /MHF2 R11A/K12A /FANCM-F K675A/K676A ), 5, 20 μM; lane 8-9 (MHF1 K73A/R74A /MHF2/FANCM-F K675A/K676A ): 5, 20 μM, respectively; lane 10 (MHF1 K73A/R74A /MHF2/FANCM-F): 20 μM. ( f ) MHF1 1−114 /MHF2/FANCM-F still binds to DNA. But the data could only be fitted in one-site-binding mode. ( g ) The DNA-binding trajectory in the MHF–FANCM-F complex. MHF1 C terminus locates in the junction of the two DNA-binding paths shown in orange strip, and the MHF1 C-terminal residues may follow a trajectory similar to that of α4 helix of NC2α shown in blue. Full size image We next determined the function of the MHF1 C terminus in the DNA-binding activity of MHF1/MHF2/FANCM-F. MHF1 1–107 /MHF2/FANCM-F still showed no DNA-binding activity (data not shown); MHF1 1–114 /MHF2/FANCM-F interacted with DNA, but it exhibited one-site-binding mode ( Fig. 6f ), implicating the disruption of the α1α1 site when the C-terminal MHF1 is removed. On the basis of the above results, we propose that the MHF–FANCM-F complex possesses two DNA-binding sites ( Fig. 6g ) and that they are not independent, but coupled by the C terminus of MHF1 and bind to DNA synergistically. The (MHF1–MHF2) 2 tetramer localizes FANCM to centromeres To determine the effect of MHF1 on FANCM localization, HeLa cells were transiently transfected to express GFP–FANCM and short interfering RNA to suppress the endogenous MHF1. As shown in Fig. 7a , GFP–FANCM locates to the centromeres in the scramble-transfected cells based on the superimposition of ACA staining with GFP–FANCM. A survey of 200 cells positively transfected revealed that majority of GFP–FANCM-expressing cells (>95%) exhibits a typical co-localization profile shown in Fig. 7a . However, the centromere localization of GFP–FANCM is diminished when MHF1 is suppressed. Less than 5% cells containing centromeric GFP–FANCM signal when MHF1 is knockdown ( n =200), suggesting that MHF1–MHF2 structural integrity is essential for localization of FANCM. 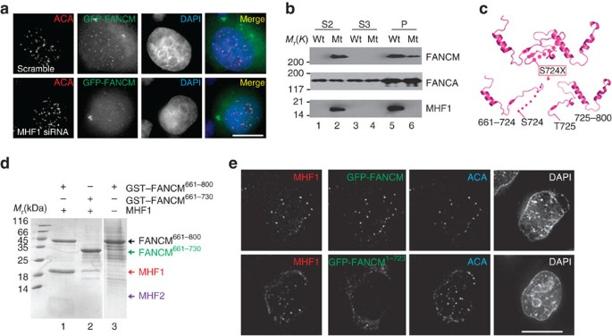Figure 7: MHF–FANCM physical contact is essential for a stable localization of FANCM to chromatin. (a) MHF1 is essential for a stable localization of FANCM to centromere. GFP–FANCM is readily apparent at the centromere in the scramble short interfering RNA-treated cells (upper panel merge). GFP–FANCM failed to localize to the centromere in the absence of MHF1 (lower panel). (b) (MHF1–MHF2)2tetramer is essential for a stable FANCM association with chromatin. (c) Schematic diagram of structure perturbation in disease-associated mutant FANCMS724X. (d) Stable MHF–FANCM-F association requires a physical contact between MHF and FANCM-F. GST pull-down results show that MHF binds to FANCM-F (FANCM661−800) (lane 1), but not FANCM661−730(lane 2). (e) Perturbation of MHF–FANCM-F association abrogates the localization of FANCM to chromatin. GFP–FANCM is readily apparent at the centromere as it co-localizes with ACA and MHF1 (upper panel). GFP–FANCM1−723failed to localize to the centromere (lower panel). Figure 7: MHF–FANCM physical contact is essential for a stable localization of FANCM to chromatin. ( a ) MHF1 is essential for a stable localization of FANCM to centromere. GFP–FANCM is readily apparent at the centromere in the scramble short interfering RNA-treated cells (upper panel merge). GFP–FANCM failed to localize to the centromere in the absence of MHF1 (lower panel). ( b ) (MHF1–MHF2) 2 tetramer is essential for a stable FANCM association with chromatin. ( c ) Schematic diagram of structure perturbation in disease-associated mutant FANCM S724X . ( d ) Stable MHF–FANCM-F association requires a physical contact between MHF and FANCM-F. GST pull-down results show that MHF binds to FANCM-F (FANCM 661−800 ) (lane 1), but not FANCM 661−730 (lane 2). ( e ) Perturbation of MHF–FANCM-F association abrogates the localization of FANCM to chromatin. GFP–FANCM is readily apparent at the centromere as it co-localizes with ACA and MHF1 (upper panel). GFP–FANCM 1−723 failed to localize to the centromere (lower panel). Full size image FANCM and MHF constitutively associate with each other in vivo [21] . To determine whether the (MHF1–MHF2) 2 tetramer is essential for a stable FANCM association with chromatin, HeLa cells were transiently transfected to express FLAG-MHF1 and FLAG-MHF1 H71A/D81A together with Myc-tagged FANCM, followed by subcellular fractionation to separate the chromatin fraction (P) from cytosolic fractions (S2 and S3) using differential centrifugation [29] . Consistent with the previously published results [29] , Myc-FANCM was exclusively detected in the chromatin fraction (P) of wild-type MHF1-expressing cells ( Fig. 7b , lane 5). FANCA distributed across the S2, S3, and P fractions of both FLAG-MHF1-expressing cells and FLAG-MHF1 H71A/D81A -expressing cells, as previously described. However, mutant MHF1 H71A/D81A was found only in the S2 fraction, consistent with our early immunofluorescence study ( Fig. 4b ), and suggesting that perturbation of the (MHF1–MHF2) 2 tetramer abolishes the association of MHF1 with chromatin. Most of myc-FANCM becomes relocated in mutant MHF1-expressing cells (for example, FLAG-MHF1 H71A/D81A -expressing cells), supporting the notion that FANCM is localized to chromatin when functional integrity of the MHF complex is present. A minor amount of myc-FANCM remains associated with chromatin faction ( Fig. 7b ; lane 6), which represents the myc-FANCM bound to the endogenous MHF complex. Localization of FANCM to chromatin Given the dependence of FANCM on the MHF complex in chromatin localization, we determined whether the disease-associated mutant FANCM S724X retains the capacity to bind the MHF complex and co-distributes with MHF to centromeres [15] . As Ser724 is situated in the top centre of the 'dual-V' shaped FANCM-F, deletion mutant near Ser724 would perturb the interaction of FANCM-F with (MHF1–MHF2) 2 ( Fig. 7c ). To this end, we performed a pull-down assay using GST–FANCM-F fusion protein, as an affinity matrix, to isolate recombinant MHF protein from bacteria. As shown in Fig. 7d , GST–FANCM-F binds tightly to MHF (lane 1). In contrast, little MHF protein binds to GST–FANCM 661–730 (lane 2). To establish that FANCM S724X perturbs its localization with MHF, we performed immunofluorescence experiments, in which HeLa cells were transiently transfected to co-express Myc-MHF1 with GFP–FANCM or GFP–FANCM 1–723 . As predicted, GFP–FANCM co-localized with Myc-MHF1 to the centromere marked by ACA ( Fig. 7e ). However, GFP–FANCM 1–723 failed to localize with Myc-MHF1 to the centromere labelled with ACA ( Fig. 7e ), which is consistent with the pull-down assay ( Fig. 7d ). These data reveal that the 'dual-V' structure of FANCM is indispensable for its association with MHF, and disruption of the 'dual-V' structure by the disease-associated mutation (S724X) causes failure in targeting of FANCM 1–723 to chromatin, which may partially explain the pathogenesis of such mutations in FA patients. In this investigation, we determined the crystal structures of the MHF1–MHF2 and MHF–FANCM-F complexes. By adopting the histone-fold motif, MHF1 and MHF2 are arranged into a tetramer, similar to the (H3–H4) 2 within histone octamers. Given the function of the MHF (CENP-S/X) complex in the assembly of kinetochores [22] , [23] , the information from our structure-functional analyses shows that plasticity of the MHF–FANCM complex is involved in maintaining genomic stability during cell division. FANCM binds to the (MHF1–MHF2) 2 tetramer, with each dimer as a subregion. The extensive interface between MHF and FANCM guards the stability of the assembled MHF–FANCM complex; thus, they translocate together to the damaged DNA site for subsequent loading and/or assembly of FA core complex [4] . The FANCM mutation S724X in FA individuals [15] would lead to truncated products of FANCM 1–723 . Our structural observations indicate that FANCM-F bears the 'dual-V' shaped configuration for physical contact with MHF. FANCM 661–730 is unable to bind to MHF, mainly because of the fact that truncation disrupts the 'dual-V' shaped configuration of FANCM-F and the interface between MHF and FANCM-F. In addition, the FANCM 1–723 deletion mutant failed to localize with MHF1 in the centromere of culture cells, suggesting that 'dual-V'-shaped FANCM forms a stable complex with the (MHF1–MHF2) 2 tetramer, which is essential for FANCM binding to chromatin. Our results provide insight into how a mutation in FANCM S724X causes mis-localization of FANCM to the chromatin. The results contribute to understanding of the etiology of FA. Given the importance of MHF in assembly of a stable MHF–FANCM to centromeres ( Fig. 7a ), the perturbation of stable MHF–FANCM complex formation by FANCM S724X may also impair the assembly of FA core complex at chromatin. Our future studies will aim to determine how the mutant FANCM alters the FA core complex activity and establish the contribution of disease-associated FANCM mutant to the pathogenesis of FA. How the MHF–FANCM complex recognizes the DNA damage ICLs, and is rapidly recruited to the damage site from the centromere site in chromatin, remains elusive. Our structural observations demonstrate that MHF and FANCM, by forming a stable complex, ensure the physical association with chromatin in vivo . The mechanism for regulation of FANCM ATPase activity and the mechanism underlying translocation of the MHF–FANCM complex along the chromatin and recognition of ICLs will require further studies at single-molecule analyses in real-time, preferably with a small molecule inhibitor. CENP-A is rapidly recruited to double-strand breaks in DNA, along with several centromeric components, such as CENP-U [30] , [31] . The centromere-targeting domain of CENP-A is necessary and sufficient for recruitment to double-strand breaks. Given the structural similarities in CENP-A and MHF and the kinetochore localization of MHF [23] , [28] , it would be of interest to determine whether MHF and CENP-A and other histones form nucleosomes in vitro and in vivo at the double-strand breaks. It would be important to know whether the MHF nucleosomes are different from the classic CENP-A-containing nucleosomes and how they interact at the double-strand breaks. Finally, it is worth noting that MHF1 and MHF2 (under the name of CENP-S and CENP-X) are constitutive components of centromere [23] , [28] . Future studies, using biophotonic tools such as FRET-based biosensors [32] , should illustrate the central questions such as the spatiotemporal dynamics of MHF1–MHF2 complex relative to CENP-A nucleosome during cell-division cycle and the functional specificity of the aforementioned complexes in DNA damage repair and kinetochore plasticity. Molecular delineation of those questions will shed light into a better understanding of the epigenetic mechanisms underlying centromere plasticity and genomic stability in mitosis [33] . Taken together, our structural and functional analyses of the MHF–FANCM-F complex have provided insights into the specificity of FANCM recognition by the (MHF1–MHF2) 2 tetramer and have advanced our understanding of the MHF–FANCM orchestration in MHF-chromatin binding. The results of this study should facilitate analyses of the molecular mechanism of replication fork surveillance and, perhaps, centromeric chromatin assembly. Cell culture HeLa and HEK293T cells were grown at 37 °C in DMEM (Invitrogen) containing 10% FBS, 100 U ml −1 penicillin, and 100 μg ml −1 streptomycin with 8% CO 2 in a humidified incubator. Recombinant protein preparation All the DNA fragments of human MHF1, MHF2 and FANCM 661–800 (FANCM-F) were amplified from a human brain complementary DNA library by PCRs. The MHF1 DNA fragment was cloned into a modified pET-28a (+) vector without the thrombin cleavage site using the Nde I/ Xho I restriction site. The DNA fragments of MHF2 and FANCM-F were inserted into another modified pET-28a (+) with a MBP–TEV cleavage site tag in the N-terminal recombinant proteins, respectively. All the mutants were generated using two-step PCR and subcloned, overexpresssed, and purified in the same way as that of wild-type protein. Overexpression of all recombinant proteins was induced in Escherichiacoli Rosetta (DE3) (Novagen) by 0.5 mM isopropyl-b-D-thiogalactoside, when the cell density reached OD 600 nm =0.6–0.8. After a growth for about 20 h at 16 °C, the cells were collected and lysed. The recombinant proteins were purified using Ni 2+ -nitrilotriacetate affinity resin (Ni-NTA, Qiagen) in 20 mM Tris-HCl, pH 8.0, and 200 mM NaCl. Then, the MBP tag in the target protein was removed by TEV digestion at 4 °C overnight. The proteins were further purified using HiTrap Q FF (5 ml) and HiLoad 16/60 Superdex 200 (GE Healthcare). The final proteins in buffer containing 20 mM Tris-HCl, pH 7.5 and 50 mM NaCl were concentrated to 40–60 mg ml −1 for crystallization trials. To prepare the SeMet-derivative protein, MHF complex was expressed in E. coli strain B834 (Novagen) using M9 medium supplemented with SeMet and six amino acids, including leucine, isoleucine, valine, phenylalanine, lysine, and threonine. The SeMet-derivative MHF protein was then copurified with native FANCM-F protein by a procedure similar to that described above. Crystallization Full-length MHF1 (1-138 aa) and the three different truncations containing residues 1-107 aa, 1-114 aa and 1-122 aa in complex with MHF2 were all subjected to crystal screens, respectively. Both MHF1 1–107 /MHF2 and MHF1 1–114 /MHF2 complex yielded crystals, but only the former one, which was grown in 0.1 M HEPES-NaOH, pH 6.8, diffracted well enough to allow data collection. The above three versions of truncated MHF in complex with FANCM-F were again used for crystal screen, respectively. The crystal of MHF1 1–114 /MHF2/FANCM-F diffracted best and then such truncation was used for subsequent SeMet-derivative protein preparation and crystal growth. Both the native and SeMet-derivative MHF–FANCM-F crystals appeared in 0.1 M Tris-HCl, pH 8.5, 0.2 M (NH4) 2 SO4 and 25% PEG3350 and grew to the maximum size in about 72 h. For MHF–FANCM-F, both native and heavy atom-derived crystals were directly flash frozen in a cold nitrogen stream at 100 K. For MHF, the crystals were co-cryoprotected in buffer containing 0.1 M HEPES-NaOH, pH 6.8 and 30% glycerol. All the crystal screen attempts were carried out using hanging drop vapour diffusion method at 285 K. Data collection and structure determination All data were collected at beamline BL17U of Shanghai Synchrotron Radiation Facility (SSRF) and processed with the HKL2000 package [34] and programs in the CCP4 suite [35] . For SeMet-derivative MHF–FANCM-F crystal, data were collected at the wavelength near the selenium absorption edge. The single wavelength anomalous scattering data of MHF–FANCM-F collected from a single SeMet-derivative crystal was enough to calculate the initial phases. The phases were calculated by PHENIX.AutoSol [36] , and a figure of merit (FOM) of 0.4 and 0.65 was acquired before and after the density modification, respectively. Then, the phase information was used to build initial model with the program PHENIX.AutoBuild [36] . The initial model was then completed through several cycles of manual model rebuilding in COOT [37] and refinement in Refmac5 (ref. 38 ). The MHF–FANCM-F complex structure was further refined to 2.64 Å, using PHENIX.refine [33] , until all the density in the map could be interpreted well and all residues have acceptable chemical confirmation with 94% of the residues falling in most favoured Ramachandran region and 6% in the allowed category. The MHF complex structure was determined by molecular replacement using Molrep [39] in the CCP4i suite [35] . The MHF dimer from the MHF–FANCM-F complex was used as the search model. The model from the Molrep was refined to the full resolution range against the native data of MHF using Refmac5 (ref. 38 ), PHENIX.refine [36] and manual rebuilding in COOT [37] . TLS restraint in the PHENIX.refine was used in the last several cycles of refinement. The final model gives 97% of residues residing in most favoured region and 3% in allowed region. All structures were checked by MolProbity [40] and figures were prepared using PyMOL (DeLano Scientific). Electrophoretic mobility shift assay DNA-binding reactions (10 μl) were carried out for 1 h at 4 °C in binding buffer (20 mM Tris-HCl, pH7.5, 50 mM NaCl) with the indicated concentration of protein and 0.6 μM DNA. After the addition of 3 μl of gel loading buffer (50% glycerol, 0.02% bromophenol blue), the reaction mixtures were resolved in 5% native polyacrylamide gel in 0.5×TBE buffer (45 mM Tris-borate, 1 mM EDTA, pH 8.0) at 4 °C for 60 min and visualized by Gel-Red-staining. The DNA probe is same to that used in fluorescence polarization assays. Fluorescence polarization assays FPAs were performed at 298 K using a SpectraMax M5 microplate reader system in buffer containing 20 mM Tris-HCl pH 7.5, 50 mM NaCl. The wavelengths of fluorescence excitation and emission were 490 nm and 522 nm, respectively. Each well of a 384-well plate contained 100 nM fluorescent-labelled (5′-FAM) DNA probe and different amounts of protein complexes with a final volume of 80 μl. For each assay, DNA-free controls were included. The fluorescence polarization P (in mP units) was calculated with the equation: P =( I i − I − )/( I i + I − ). The fluorescence polarization change P (in mP units) was fit to the equation Δ P = P max × [protein]/( K d + [protein]) for one-site-bind mode and equation for two-site-bind mode. The dsDNA probe used in the assays was formed by annealing ssDNA with complementary ssDNA. The sequence of single-strand DNA (ssDNA) was: 5′-ACGCTGCCGAATTCTACCAGTGCCTTGCTAGGACATCTTTGCCCACCTGCAGGTTCACC-3′. GST-pull-down assays A similar amount of purified MHF complex was added to a similar amount of E. coli cells expressing recombinant GST–FANCM-F (GST–FANCM 661–800 ) or GST–FANCM 661–730 , and then the mixtures were lysed in buffer containing 20 mM Tris-HCl pH 7.5, 200 mM NaCl. The supernatant was incubated with 100 μl of GST beads for 30 min at room temperature. Then, the beads were washed two times with binding buffer. Finally, the bound proteins eluted from the beads were resolved by SDS–PAGE (15%) and stained with Coomassie brilliant blue (BioRad, USA). Immunofluorescence microscopy Aliquots of HeLa cells were transiently transfected to express MHF1, MHF2 and their mutants using Lipofectamine 2000 as previously described [41] . Twenty-four hours after transfection, cells on glass coverslips were washed with warm PHEM (60 mM PIPES, 25 mM HEPES, 10 mM EGTA, 2 mM MgCl 2 , pH 6.9), followed by 1 min of permeabilization with PHEM containing 0.1% Triton X-100 at 37 °C followed by fixation in 3.7% paraformaldehyde for 5 min. After being washed three times with PBS, cells were blocked with 1% bovine serum albumin (BSA, Sigma) in PBS containing 0.5% Tween-20 for 30 min, then incubated with primary antibodies for 1 h, followed by secondary antibodies for 45 min. DNA was stained with 4′,6-diamidino-2-phenylindole (DAPI, 1:10,000, Sigma) and human ACA (1:500) [42] . Secondary antibodies were purchased from Invitrogen and used at a concentration of 1:400. Images were acquired every 0.25 μm at z -axis to generate three-dimensional image stacks utilizing an Olympus 60X/1.42 Plan APO N objective on an Olympus IX71 microscope (Applied Precision DeltaVision Personal). The three- image stacks were de-convolved, projected with SoftWorx (Applied Precision), and mounted in figures with Adobe Photoshop and Illustrator (Adobe) [43] . Accession codes: Atomic coordinates and structure factors for the MHF1–MHF2 and MHF–FANCM complex have been deposited in the Protein Data Bank under the accession codes 4DRA and 4DRB , respectively. How to cite this article: Tao, Y. et al . The structure of the FANCM–MHF complex reveals physical features for functional assembly. Nat. Commun. 3:782 doi: 10.1038/ncomms1779 (2012).